Simultaneous downregulation of KLF5 and Fli1 is a key feature underlying systemic sclerosis Systemic sclerosis (SSc) is manifested by fibrosis, vasculopathy and immune dysregulation. So far, a unifying hypothesis underpinning these pathological events remains unknown. Given that SSc is a multifactorial disease caused by both genetic and environmental factors, we focus on the two transcription factors, which modulate the fibrotic reaction and are epigenetically suppressed in SSc dermal fibroblasts, Friend leukaemia integration 1 (Fli1) and Krüppel-like factor 5 (KLF5). In addition to the Fli1 silencing-dependent collagen induction, the simultaneous knockdown of Fli1 and KLF5 synergistically enhances expression of connective tissue growth factor. Notably, mice with double heterozygous deficiency of Klf5 and Fli1 mimicking the epigenetic phenotype of SSc skin spontaneously recapitulate all the three features of SSc, including fibrosis and vasculopathy of the skin and lung, B-cell activation and autoantibody production. These studies implicate the epigenetic downregulation of Fli1 and KLF5 as a central event triggering the pathogenic triad of SSc. Systemic sclerosis (SSc) is a multisystem chronic disease characterized by three major abnormalities, including vasculopathy, immune dysregulation and fibrosis of the skin and certain internal organs, especially lungs [1] . Vasculopathy is recognized as structural damage of small vessels, reduced blood flow and subsequent tissue hypoxia, leading to skin ulcers and pulmonary hypertension. Immune dysregulation is characterized by autoantibody production, abnormally activated immune cells and release of various cytokines. Transforming growth factor-β (TGF-β) and connective tissue growth factor (CTGF or CCN2) are widely recognized as key fibrotic mediators in SSc [2] , [3] , [4] , whose coadministration is sufficient to induce persistent fibrosis in mouse models [5] , [6] . So far, a unifying hypothesis underpinning the three major abnormalities of SSc remains unknown, which prevents the understanding of its pathogenesis and the development of ideal therapy. Lack of mouse models with all three features has also hindered this research. SSc is a multifactorial disease caused by the complex interplay between hereditary and environmental factors. Friend leukaemia integration 1 (Fli1), a member of the Ets transcription factor family, is a potent repressor of the type I collagen gene and mediates a non-canonical pathway of TGF-β [7] . Epigenetic downregulation of Fli1 in patient dermal fibroblasts is potentially involved in the fibrotic processes of SSc by partially mimicking TGF-β stimulation [8] . However, Fli1 +/− mice do not develop clinically apparent dermal fibrosis, implying a contribution of additional factors besides Fli1 deficiency to the development of SSc. Through an extensive literature search, we noted that Krüppel-like factor 5 (KLF5), a member of the SP/KLF transcription factor family [9] , may be a potential additional factor. KLF5 gene expression is downregulated in SSc skin [4] and Klf5 haploinsufficiency alters the fibrotic response following experimental tissue damage in the heart and kidney [10] , [11] . Although mice with homozygous deletion of Klf5 or Fli1 die in utero [12] , [13] , we found that mice with double heterozygous deficiency of Klf5 and Fli1 spontaneously develop tissue fibrosis, vasculopathy, B-cell activation and autoantibody production, which are quite similar to those of SSc. Vascular injury and autoantibody production have been considered as the earliest and possibly primary events in SSc [1] , but this issue remains to be controversial. Our findings suggest that the downregulation of these two transcription factors may be the primary event initiating the three manifestations of SSc. Overall, the major impact of this study is the identification of the two transcription factors, KLF5 and Fli1, whose simultaneous decrease potentially underlies the development of the three major features of SSc, including autoimmunity, vasculopathy and fibrosis. This type of concept has never been suggested before, thus provoking a paradigm shift in the understanding of SSc pathogenesis. Epigenetic downregulation of KLF5 in SSc fibroblasts Immunohistochemistry, immunoblotting and quantitative reverse transcription PCR (qRT-PCR) using human skin samples and/or cultured dermal fibroblasts revealed that KLF5 expression is significantly decreased in SSc fibroblasts compared with normal fibroblasts ( Fig. 1a–d ). Several recent reports have suggested that extracellular matrix (ECM) overproduction in SSc is affected by epigenetic modifications [8] , [14] , [15] . Generally speaking, histone acetylation promotes gene expression and DNA methylation represses gene transcription [16] . To investigate whether KLF5 expression is epigenetically inhibited in SSc fibroblasts, cultured fibroblasts were treated with two epigenetic inhibitors, 5-aza-2′-deoxycytidine (a DNA methyltransferase inhibitor) and trichostatin A (a histone deacetylase inhibitor), leading to an over threefold increase in KLF5 expression and a 50% decrease in COL1A2 expression in SSc fibroblasts without effect on normal fibroblasts ( Fig. 1e ). As for histone acetylation, chromatin immunoprecipitation (ChIP) indicated that histone H3 and H4 on the KLF5 promoter were significantly less acetylated in SSc fibroblasts than in normal fibroblasts ( Fig. 1f ). Furthermore, regarding DNA methylation, bisulfite sequencing revealed that certain CpG islands in the KLF5 promoter were partly methylated in SSc fibroblasts, while they were completely unmethylated in normal fibroblasts ( Fig. 1g ). To explore whether DNA methylation alone impacts on KLF5 expression, we treated SSc fibroblasts with 5-aza-2′-deoxycytidine, resulting in an 86% increase in KLF5 expression ( Fig. 1h ). These results suggest that KLF5 expression is epigenetically suppressed in SSc fibroblasts. 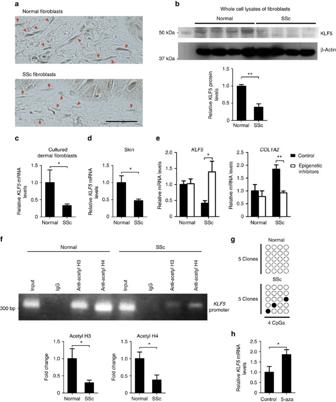Figure 1:KLF5expression is epigenetically suppressed in fibroblasts from SSc patients. (a) KLF5 staining in human skin. Arrowheads demonstrate dermal fibroblasts. Scale bar, 25 μm. (b) The representative image of KLF5 protein expression in cultured dermal fibroblasts. The result of densitometric analyses is also shown.n=4 individuals per group. Another group of three SSc and three control samples showed similar results. (c)KLF5mRNA expression in cultured dermal fibroblasts.n=5 (controls) and 8 (SSc). (d)KLF5mRNA expression in skin tissues.n=8 individuals per group. (e) Cultured dermal fibroblasts were treated with two epigenetic inhibitors, 5-aza-2′-deoxycytidine (5-aza; 5 μM) and trichostatin A (2 μM) for 48 h. mRNA levels of indicated genes were assessed.n=5 individuals per group. (f) ChIP was performed using anti-acetyl histone H3 or H4 antibodies on samples from cultured fibroblasts. PCR was performed usingKLF5proximal promoter-specific primers. The representative image and results analysed by qRT-PCR are shown. Ratios to input values were compared.n=5 individuals per group. (g) CpG islands of theKLF5proximal promoter. Filled circles indicate methylated CpG sites and open circles demonstrate unmethylated CpG sites. The amplicon contains four CpG sites extending from −273 to −210 bp of the transcription start site. Five clones were examined for each patient. The representative data from four SSc patients and four normal individuals are shown. (h)KLF5mRNA levels were assessed in fibroblasts treated with 5-aza (5 μM) for 48 h.n=5 individuals per group. Data are mean±s.e.m. *P<0.05, **P<0.01 by two-tailed unpairedt-test. Figure 1: KLF5 expression is epigenetically suppressed in fibroblasts from SSc patients. ( a ) KLF5 staining in human skin. Arrowheads demonstrate dermal fibroblasts. Scale bar, 25 μm. ( b ) The representative image of KLF5 protein expression in cultured dermal fibroblasts. The result of densitometric analyses is also shown. n =4 individuals per group. Another group of three SSc and three control samples showed similar results. ( c ) KLF5 mRNA expression in cultured dermal fibroblasts. n =5 (controls) and 8 (SSc). ( d ) KLF5 mRNA expression in skin tissues. n =8 individuals per group. ( e ) Cultured dermal fibroblasts were treated with two epigenetic inhibitors, 5-aza-2′-deoxycytidine (5-aza; 5 μM) and trichostatin A (2 μM) for 48 h. mRNA levels of indicated genes were assessed. n =5 individuals per group. ( f ) ChIP was performed using anti-acetyl histone H3 or H4 antibodies on samples from cultured fibroblasts. PCR was performed using KLF5 proximal promoter-specific primers. The representative image and results analysed by qRT-PCR are shown. Ratios to input values were compared. n =5 individuals per group. ( g ) CpG islands of the KLF5 proximal promoter. Filled circles indicate methylated CpG sites and open circles demonstrate unmethylated CpG sites. The amplicon contains four CpG sites extending from −273 to −210 bp of the transcription start site. Five clones were examined for each patient. The representative data from four SSc patients and four normal individuals are shown. ( h ) KLF5 mRNA levels were assessed in fibroblasts treated with 5-aza (5 μM) for 48 h. n =5 individuals per group. Data are mean±s.e.m. * P <0.05, ** P <0.01 by two-tailed unpaired t -test. Full size image Klf5 heterozygosity augments skin fibrotic responses We then assessed the in vivo function of KLF5 using a mouse model of bleomycin-induced dermal fibrosis [17] . Compared with bleomycin-challenged wild-type (WT) mice, bleomycin-treated Klf5 +/− mice showed greater levels of dermal thickness, myofibroblast and CTGF-positive fibroblast counts, and Ctgf and Col1a2 mRNA expression, while these parameters were comparable after PBS injection ( Fig. 2a–e ). Furthermore, while dermal thickness in WT mice significantly decreased during a 3-month observation period after the completion of bleomycin injections, bleomycin-challenged Klf5 +/− mice did not lose dermal thickness ( Supplementary Fig. 1a,b ). When crossing Tsk/+ mice with Klf5 +/− mice to investigate the impact of Klf5 heterozygosity in a less inflammatory fibrotic model [18] , compared with Tsk/+ mice, Tsk/+ ; Klf5 +/− mice showed higher levels of hypodermal thickness, myofibroblast and CTGF-positive fibroblast counts, and Ctgf and Col1a2 mRNA expression ( Supplementary Fig. 2a–e ). To determine the contribution of fibroblast KLF5 deficiency to the observed cutaneous phenotypes in Klf5 +/− mice, we selectively ablated Klf5 gene in fibroblasts by crossing Klf5 floxed mice ( Klf5 fl/fl ) with Col1a2-Cre/ERT mice and administering tamoxifen intraperitoneally. On BLM challenge, Klf5 fl/fl ; Col1a2-Cre/ERT mice demonstrated fibrosis-prone skin phenotypes similar to Klf5 +/− mice ( Supplementary Fig. 3a–f ). These results indicate that Klf5 deficiency contributes to the development and maintenance of skin fibrosis when pro-fibrotic microenvironment, such as bleomycin challenge and Tsk/+ phenotype, is present. 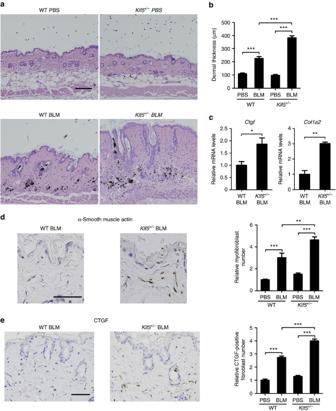Figure 2:Klf5heterozygous deficiency exacerbates bleomycin (BLM)-induced dermal fibrosis. Subcutaneous injections of BLM (300 μg every other day for 3 weeks) were given to the back skin of female mice at 6 weeks of age. (a) Representative skin sections of WT andKlf5+/−mice injected with PBS or BLM. Scale bar, 100 μm. (b) Dermal thickness of each group is summarized.n=4 mice per group. (c) mRNA expression ofCtgfandCol1a2in the skin tissue assessed by qRT-PCR.n=3 mice per group. (d,e) The relative numbers of myofibroblasts (d) and CTGF-positive fibroblasts (e) in the dermis. The number per high power field is adjusted to that in PBS-treated WT mice set at 1. The representative pictures of skin histology in WT andKlf5+/−mice treated with BLM are also shown. Scale bar, 50 μm.n=4 mice per group. Data are mean±s.e.m. *P<0.05, **P<0.01, ***P<0.001 by one-way ANOVA with Bonferroni’spost hoctest forb,d,eand two-tailed unpairedt-test forc. One additional independent experiment using another group of mice provided similar results. Figure 2: Klf5 heterozygous deficiency exacerbates bleomycin (BLM)-induced dermal fibrosis. Subcutaneous injections of BLM (300 μg every other day for 3 weeks) were given to the back skin of female mice at 6 weeks of age. ( a ) Representative skin sections of WT and Klf5 +/− mice injected with PBS or BLM. Scale bar, 100 μm. ( b ) Dermal thickness of each group is summarized. n =4 mice per group. ( c ) mRNA expression of Ctgf and Col1a2 in the skin tissue assessed by qRT-PCR. n =3 mice per group. ( d , e ) The relative numbers of myofibroblasts ( d ) and CTGF-positive fibroblasts ( e ) in the dermis. The number per high power field is adjusted to that in PBS-treated WT mice set at 1. The representative pictures of skin histology in WT and Klf5 +/− mice treated with BLM are also shown. Scale bar, 50 μm. n =4 mice per group. Data are mean±s.e.m. * P <0.05, ** P <0.01, *** P <0.001 by one-way ANOVA with Bonferroni’s post hoc test for b , d , e and two-tailed unpaired t -test for c . One additional independent experiment using another group of mice provided similar results. Full size image KLF5 transcriptionally represses CTGF gene expression To further explore the mechanism of the exaggerated fibrotic response under Klf5 heterozygous deficiency, we assessed the mRNA levels of fibrosis-associated molecules using cultured dermal fibroblasts, which identified 50% increased Ctgf mRNA levels in Klf5 +/− fibroblasts compared with WT fibroblasts, while the levels of other fibrotic markers, Col1a2 , Acta2 (encoding α-smooth muscle actin, α-SMA), and Itgb5 (encoding integrin β5), were comparable ( Supplementary Fig. 4 ). Human foreskin fibroblasts transfected with small interfering RNA (siRNA) against KLF5 also demonstrated an increase in CTGF mRNA and protein levels both at the basal state and under TGF-β1 stimulation ( Fig. 3a,b ). Furthermore, KLF5 overexpression decreased CTGF reporter activity maximally by 65% in a dose-dependent manner ( Fig. 3c ), while KLF5 gene silencing increased CTGF reporter activity by 49% ( Fig. 3d ). 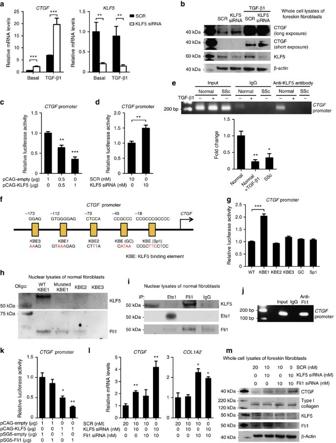Figure 3: KLF5 and Fli1 coordinately repressCTGFtranscription. (a,b) Foreskin fibroblasts were transfected with scrambled control RNA (SCR) or KLF5 siRNA for 24 h and stimulated with TGF-β1 (2 ng ml−1) for an additional 24 h under serum starvation. Expression levels were assessed by qRT-PCR (a) and immunoblotting (b). (c,d) Luciferase assays usingCTGFpromoter constructs. Foreskin fibroblasts were cotransfected with indicated vectors (c) or with SCR or KLF5 siRNA (d). Thirty hours after transfection, luciferase activity was measured. (e) ChIP on fibroblasts was performed using anti-KLF5 antibodies and primers specific for the KLF5-binding site on theCTGFpromoter. The results of qRT-PCR normalized to input values are summarized.n=4 individuals per group. (f) Putative KLF5-binding sites on theCTGFpromoter and mutated sequences (red letters). KBE, KLF5-binding element. (g) Luciferase assays performed as incusing mutated promoter constructs. (h) Oligonucleotide pull-down assays using oligonucleotides containing KBE1 with or without mutation, KBE2 and KBE3. Input corresponds with fibroblast nuclear lysates before oligonucleotide binding. Oligo, oligonucleotides. (i) Fibroblast nuclear extracts were immunoprecipitated and blotted with indicated antibodies. IP, immunoprecipitation. (j) ChIP on fibroblasts was performed using anti-Fli1 antibodies and primers specific for the KLF5-binding site on theCTGFpromoter. (k) Luciferase assays performed as inc. (l,m) Fibroblasts were treated with SCR or indicated siRNA for 24 h and serum starved for 24 h. mRNA levels (l) and protein levels (m) were assessed. Data are mean±s.e.m. of three independent experiments. Blotting results are representatives of three independent experiments. *P<0.05, **P<0.01, ***P<0.001 by two-tailed unpairedt-test. Significant differences inc,e,g,k,lare compared with the leftmost group. Figure 3: KLF5 and Fli1 coordinately repress CTGF transcription. ( a , b ) Foreskin fibroblasts were transfected with scrambled control RNA (SCR) or KLF5 siRNA for 24 h and stimulated with TGF-β1 (2 ng ml −1 ) for an additional 24 h under serum starvation. Expression levels were assessed by qRT-PCR ( a ) and immunoblotting ( b ). ( c , d ) Luciferase assays using CTGF promoter constructs. Foreskin fibroblasts were cotransfected with indicated vectors ( c ) or with SCR or KLF5 siRNA ( d ). Thirty hours after transfection, luciferase activity was measured. ( e ) ChIP on fibroblasts was performed using anti-KLF5 antibodies and primers specific for the KLF5-binding site on the CTGF promoter. The results of qRT-PCR normalized to input values are summarized. n =4 individuals per group. ( f ) Putative KLF5-binding sites on the CTGF promoter and mutated sequences (red letters). KBE, KLF5-binding element. ( g ) Luciferase assays performed as in c using mutated promoter constructs. ( h ) Oligonucleotide pull-down assays using oligonucleotides containing KBE1 with or without mutation, KBE2 and KBE3. Input corresponds with fibroblast nuclear lysates before oligonucleotide binding. Oligo, oligonucleotides. ( i ) Fibroblast nuclear extracts were immunoprecipitated and blotted with indicated antibodies. IP, immunoprecipitation. ( j ) ChIP on fibroblasts was performed using anti-Fli1 antibodies and primers specific for the KLF5-binding site on the CTGF promoter. ( k ) Luciferase assays performed as in c . ( l , m ) Fibroblasts were treated with SCR or indicated siRNA for 24 h and serum starved for 24 h. mRNA levels ( l ) and protein levels ( m ) were assessed. Data are mean±s.e.m. of three independent experiments. Blotting results are representatives of three independent experiments. * P <0.05, ** P <0.01, *** P <0.001 by two-tailed unpaired t -test. Significant differences in c , e , g , k , l are compared with the leftmost group. Full size image To assess the interaction between KLF5 and the CTGF promoter, we performed ChIP using cultured dermal fibroblasts, showing that KLF5 binds to the CTGF promoter and that its affinity is significantly reduced in SSc fibroblasts and in TGF-β1-stimulated normal fibroblasts compared with unstimulated normal fibroblasts ( Fig. 3e ). Therefore, we individually mutated five putative KLF5-binding sites in the CTGF proximal promoter and examined their contribution to the repression of CTGF transcriptional activity ( Fig. 3f ), revealing that a mutation in the KLF-binding element 1 (KBE1; −112 to −105 bp of the transcription start site) enhances CTGF promoter activity by 2.0 folds ( Fig. 3g ). To prove that KLF5 exerts its repressive function against the CTGF promoter by binding to KBE1, we performed oligonucleotide pull down, which showed that the KBE1 mutation abrogates KLF5 binding to this sequence and also that KLF5 does not bind to KBE2 or KBE3 ( Fig. 3h ). These results demonstrate that KLF5 represses CTGF transcriptional activity by binding to a specific promoter region. KLF5 and Fli1 synergistically repress CTGF transcription Two of the Ets family members, Ets1 and Fli1, bind to a site close to KBE1, within −126 to −77 bp of the CTGF promoter [19] , [20] . Therefore, we investigated whether KLF5 interacts with Ets1 or Fli1. Immunoprecipitation detected that KLF5 physically interacts with Fli1, but not with Ets1 ( Fig. 3i ). We also confirmed the binding of Fli1 to the CTGF promoter using ChIP ( Fig. 3j ). We further demonstrated that Fli1 binds to the KBE1 site and that this binding is significantly attenuated when this site is mutated ( Fig. 3h ). Thus, the Fli1/KLF5 complex binds to the KBE1 region of the CTGF promoter and both factors dissociate from KBE1 when KLF5 binding to KBE1 is lost. To explore whether KLF5 and Fli1 cooperatively regulate CTGF transcription, we cotransfected human foreskin fibroblasts with KLF5 and Fli1 expression vectors. While Fli1 overexpression alone only marginally suppressed CTGF transcription, it synergistically enhanced the inhibitory function of KLF5 ( Fig. 3k ). Consistently, simultaneous gene silencing of KLF5 and FLI1 synergistically increased CTGF levels, while KLF5 downregulation did not affect type I collagen expression, which is regulated by Fli1 (ref. 7 ) ( Fig. 3l,m ). We further confirmed that CTGF expression is enhanced proportionally to the downregulation of the two transcription factors, suggesting that CTGF gene expression is regulated directly by KLF5 and Fli1 rather than by a paradoxical activation of other signalling pathways ( Supplementary Fig. 5 ). These results indicate that KLF5 and Fli1 form a transcriptional complex on the CTGF promoter and negatively regulate its transcriptional activity. Downregulation of KLF5 and Fli1 is a hallmark of SSc The data described above suggested that the simultaneous downregulation of KLF5 and Fli1 might be a molecular hallmark of SSc dermal fibroblasts, particularly explaining the overexpression of CTGF in those cells. To further confirm this notion, we immunohistochemically investigated the expression of KLF5 and Fli1 in SSc dermal fibroblasts obtained from patients with the three representative autoantibody patterns (anti-topoisomerase I, anti-centromere and anti-RNA polymerase III antibodies). SSc patients positive for anti-topoisomerase I antibody or anti-centromere antibody demonstrated significant downregulation of both KLF5 and Fli1 in dermal fibroblasts compared with healthy controls ( Fig. 4a,b ). In SSc patients with anti-RNA polymerase III antibody, the extent of downregulation was smaller than in SSc patients with the other two antibodies. Importantly, when we evaluated whether KLF5 expression parallels that of Fli1 in SSc skin, the levels of KLF5 and Fli1 mRNAs showed significant positive correlation ( r =0.88, P =0.033; two-tailed Spearman’s correlation; Fig. 4c ). We also examined the expression patterns of the two transcription factors in the skin of patients with other fibrotic diseases. KLF5 and Fli1 showed remarkable downregulation in morphea, while Fli1-selective downregulation was observed in eosinophilic fasciitis. These results indicate that simultaneous downregulation of KLF5 and Fli1 is a molecular hallmark of SSc dermal fibroblasts. 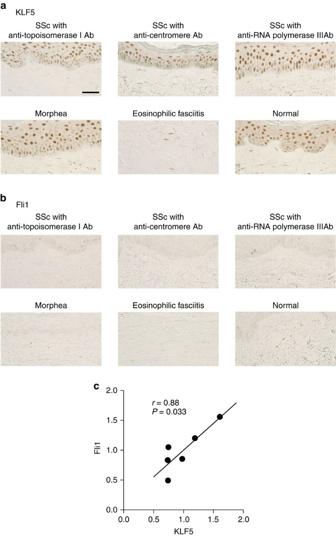Figure 4: Simultaneous downregulation of KLF5 and Fli1 is a molecular hallmark of SSc dermal fibroblasts. (a,b) Dermal fibroblasts have distinct expression patterns with KLF5 and Fli1 staining in a variety of fibrotic diseases. Representative pictures fromn=5 individuals per group are shown. (a) KLF5 staining. (b) Fli1 staining. Scale bar, 50 μm. (c) Correlation between KLF5 and Fli1 mRNA expression levels in cultured fibroblasts from SSc patients. KLF5 and Fli1 expressions were quantified by qRT-PCR. Samples from six dcSSc patients were used. Five were positive for anti-topoisomerase I antibody and one was negative for ANA. Ab, antibody. Figure 4: Simultaneous downregulation of KLF5 and Fli1 is a molecular hallmark of SSc dermal fibroblasts. ( a , b ) Dermal fibroblasts have distinct expression patterns with KLF5 and Fli1 staining in a variety of fibrotic diseases. Representative pictures from n =5 individuals per group are shown. ( a ) KLF5 staining. ( b ) Fli1 staining. Scale bar, 50 μm. ( c ) Correlation between KLF5 and Fli1 mRNA expression levels in cultured fibroblasts from SSc patients. KLF5 and Fli1 expressions were quantified by qRT-PCR. Samples from six dcSSc patients were used. Five were positive for anti-topoisomerase I antibody and one was negative for ANA. Ab, antibody. Full size image Klf5 +/− ; Fli1 +/− mice spontaneously develop dermal fibrosis Since in human SSc samples, KLF5 and Fli1 expression is downregulated but not completely absent, we sought to mimic the defects by using Klf5 +/− ; Fli1 +/− mice. Klf5 +/− ; Fli1 +/− mice were fertile, born in Mendelian ratio and did not display any apparent early developmental abnormalities. In Klf5 +/− ; Fli1 +/− mice, KLF5 and Fli1 levels were reduced to about a half of those in WT mice in the skin, lung and cultured dermal fibroblasts ( Supplementary Fig. 6a–c and Fig. 7i,j ). Strikingly, the dermis was thicker by 45% and collagen fibres were more tightly packed in 3-month-old Klf5 +/− ; Fli1 +/− mice than in WT mice ( Fig. 5a–c ), while these changes were not apparent in 2-month-old Klf5 +/− ; Fli1 +/− mice. Moreover, the skin of Klf5 +/− ; Fli1 +/− mice, in contrast to that of Klf5 +/− or Fli1 +/− mice ( Supplementary Fig. 7a–c ), demonstrated higher levels of total collagen content, mRNA expression of pro-fibrotic marker genes and myofibroblast and CTGF-positive fibroblast counts ( Fig. 5d–g ). To determine which signalling pathway is mainly involved in the fibrotic process in Klf5 +/− ; Fli1 +/− mice, we cultured Klf5 +/− ; Fli1 +/− dermal fibroblasts and assessed the activation status of canonical and non-canonical TGF-β signalling. Heterozygosity of KLF5 and Fli1 induced the phosphorylation of Smad3, ERK, p38 and JNK ( Fig. 5h ), indicating that both canonical and non-canonical TGF-β pathways are activated in Klf5 +/− ; Fli1 +/− skin. Given that coadministration of TGF-β and CTGF is sufficient to induce persistent fibrosis in mouse models [5] , [6] , our results suggest that upregulation of ECM genes due to Fli1 reduction, which mimics TGF-β stimulation, in combination with CTGF overproduction induced by simultaneous downregulation of KLF5 and Fli1 leads to spontaneous dermal fibrosis in Klf5 +/− ; Fli1 +/− mice, which largely recapitulates the molecular signature of SSc patients. 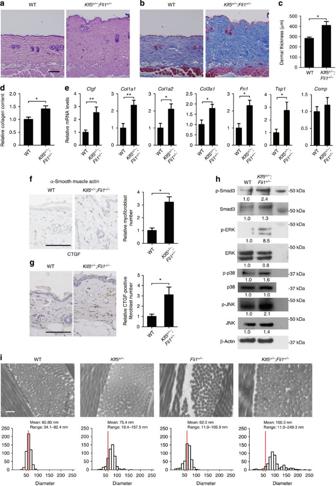Figure 5:Klf5+/−;Fli1+/−mice spontaneously develop dermal fibrosis. Skin histology in 3-month-old male mice with haematoxylin and eosin staining (a) and Masson’s trichrome staining (b). Scale bar, 100 μm. (c) Dermal thickness is summarized.n=7 male mice per group. (d) Relative skin collagen content.n=8 mice per group. (e) mRNA levels of ECM proteins in the skin are assessed by qRT-PCR.n=8 mice per group. (f,g) The relative numbers of myofibroblasts (f) and CTGF-positive fibroblasts (g).n=5 mice per group. Scale bar, 100 μm. (h) Immunoblotting for molecules related to canonical and non-canonical TGF-β pathways in dermal fibroblasts. Relative densitometric values are shown below the bands. (i) Collagen fibril alignment in the superficial dermis was examined by transmission electron microscopy. Scale bar, 200 nm. Frequency distribution profiles were obtained by measuring 500 collagen fibrils. Red bars show the diameter most frequently seen in WT mice. Data are mean±s.e.m. *P<0.05, **P<0.01 by two-tailed Mann–WhitneyU-test. Figure 5: Klf5 +/− ; Fli1 +/− mice spontaneously develop dermal fibrosis. Skin histology in 3-month-old male mice with haematoxylin and eosin staining ( a ) and Masson’s trichrome staining ( b ). Scale bar, 100 μm. ( c ) Dermal thickness is summarized. n =7 male mice per group. ( d ) Relative skin collagen content. n =8 mice per group. ( e ) mRNA levels of ECM proteins in the skin are assessed by qRT-PCR. n =8 mice per group. ( f , g ) The relative numbers of myofibroblasts ( f ) and CTGF-positive fibroblasts ( g ). n =5 mice per group. Scale bar, 100 μm. ( h ) Immunoblotting for molecules related to canonical and non-canonical TGF-β pathways in dermal fibroblasts. Relative densitometric values are shown below the bands. ( i ) Collagen fibril alignment in the superficial dermis was examined by transmission electron microscopy. Scale bar, 200 nm. Frequency distribution profiles were obtained by measuring 500 collagen fibrils. Red bars show the diameter most frequently seen in WT mice. Data are mean±s.e.m. * P <0.05, ** P <0.01 by two-tailed Mann–Whitney U -test. 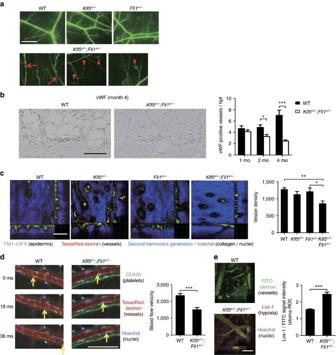Figure 6:Klf5+/−;Fli1+/−mice demonstrate vascular abnormalities in the skin. (a) Cutaneous vasculature visualized by FITC-conjugated dextran in 2-month-old-mice. Arrows show vascular stenosis and arrowheads demonstrate bushy capillary tips. Scale bar, 300 μm. The representative images fromn=4 mice per group. (b) The number of subcutaneous vessels was determined by von Willebrand factor (vWF) staining. Representative images are shown. Scale bar, 100 μm.n=15 high power fields (h.p.f.) from three mice per time point. (c–e)In vivoimaging visualizes the skin of 4-month-old male mice with indicated three colours. (c) Horizontal sections and longitudinal sections of dermis. Vessel density is quantified.n=20 fields from four mice per group. Scale bar, 100 μm. (d) Cutaneous arterioles. The arrows show flowing leukocytes at every 18-ms interval. Arteriolar blood velocities are calculated.n=15 fields from three mice per group. Scale bar, 100 μm. (e) Interstitial hypoxia measured by hypoxia probe (Lox-1) in 4-month-old-mice.n=20 fields from four mice per group. Scale bar, 100 μm. Data are mean±s.e.m. *P<0.05, **P<0.01, ***P<0.001 by two-tailed Mann–WhitneyU-test except forcwith one-way analysis of variance with Bonferroni’spost hoctest. Full size image Figure 6: Klf5 +/− ; Fli1 +/− mice demonstrate vascular abnormalities in the skin. ( a ) Cutaneous vasculature visualized by FITC-conjugated dextran in 2-month-old-mice. Arrows show vascular stenosis and arrowheads demonstrate bushy capillary tips. Scale bar, 300 μm. The representative images from n =4 mice per group. ( b ) The number of subcutaneous vessels was determined by von Willebrand factor (vWF) staining. Representative images are shown. Scale bar, 100 μm. n =15 high power fields (h.p.f.) from three mice per time point. ( c – e ) In vivo imaging visualizes the skin of 4-month-old male mice with indicated three colours. ( c ) Horizontal sections and longitudinal sections of dermis. Vessel density is quantified. n =20 fields from four mice per group. Scale bar, 100 μm. ( d ) Cutaneous arterioles. The arrows show flowing leukocytes at every 18-ms interval. Arteriolar blood velocities are calculated. n =15 fields from three mice per group. Scale bar, 100 μm. ( e ) Interstitial hypoxia measured by hypoxia probe (Lox-1) in 4-month-old-mice. n =20 fields from four mice per group. Scale bar, 100 μm. Data are mean±s.e.m. * P <0.05, ** P <0.01, *** P <0.001 by two-tailed Mann–Whitney U -test except for c with one-way analysis of variance with Bonferroni’s post hoc test. 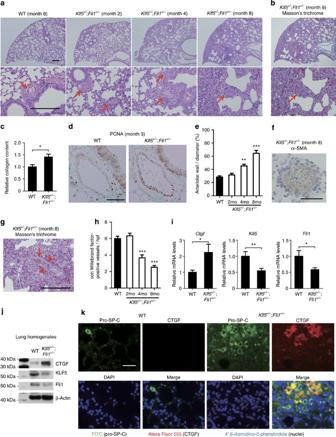Figure 7:Klf5+/−;Fli1+/−mice demonstrate interstitial lung fibrosis and vascular occlusions. (a) Lung histopathology with haematoxylin and eosin staining (a) and Masson’s trichrome staining (b). Scale bar, 200 μm. Arrows show bronchiolar arterioles. (c) Relative lung collagen content.n=4 mice per group. (d) Proliferating cell nuclear antigen (PCNA) staining of bronchiolar arterioles in WT andKlf5+/−;Fli1+/−mice. Scale bar, 50 μm. A: arteriole. B: bronchiole. (e) Quantification of arteriolar stenosis.n=15 vessels from three mice per time point. (f) The representative occluded bronchiolar arterioles in 8-month-oldKlf5+/−;Fli1+/−mice with α-SMA staining. Scale bar, 50 μm. (g) The representative interseptal venule of 8-month-oldKlf5+/−;Fli1+/−mice with Masson’s trichrome staining. Arrowheads show luminal narrowing. An arrow shows erythrocyte congestion. Scale bar, 200 μm. (h) The number of capillaries was determined by immunohistochemical staining for the endothelial cell marker, von Willebrand factor (vWF), in lung sections.n=15 high power fields (h.p.f.) from three mice per time point. (i)Ctgf,Klf5andFli1mRNA levels in the lung were assessed by qRT-PCR.n=9 mice per group. (j) Protein levels of CTGF, KLF5 and Fli1 in lung homogenates were assessed by immunoblotting. The results are from representative experiments that have been repeated three times in different pairs of mice with similar results. (k) Representative lung sections from three WT and threeKlf5+/−;Fli1+/−mice are shown. Pro-surfactant protein C (pro-SP-C), a specific marker for type 2 alveolar cells, is stained with FITC (green). CTGF is stained with Alexa Flour 555 (red). Nuclei are stained with 4′,6-diamidino-2-phenylindole (DAPI, blue). Scale bar, 50 μm. Data are mean±s.e.m. *P<0.05, **P<0.01, ***P<0.001 by two-tailed Mann–WhitneyU-test. The significant differences ine,hare compared with WT groups. Full size image Figure 7: Klf5 +/− ; Fli1 +/− mice demonstrate interstitial lung fibrosis and vascular occlusions. ( a ) Lung histopathology with haematoxylin and eosin staining ( a ) and Masson’s trichrome staining ( b ). Scale bar, 200 μm. Arrows show bronchiolar arterioles. ( c ) Relative lung collagen content. n =4 mice per group. ( d ) Proliferating cell nuclear antigen (PCNA) staining of bronchiolar arterioles in WT and Klf5 +/− ; Fli1 +/− mice. Scale bar, 50 μm. A: arteriole. B: bronchiole. ( e ) Quantification of arteriolar stenosis. n =15 vessels from three mice per time point. ( f ) The representative occluded bronchiolar arterioles in 8-month-old Klf5 +/− ; Fli1 +/− mice with α-SMA staining. Scale bar, 50 μm. ( g ) The representative interseptal venule of 8-month-old Klf5 +/− ; Fli1 +/− mice with Masson’s trichrome staining. Arrowheads show luminal narrowing. An arrow shows erythrocyte congestion. Scale bar, 200 μm. ( h ) The number of capillaries was determined by immunohistochemical staining for the endothelial cell marker, von Willebrand factor (vWF), in lung sections. n =15 high power fields (h.p.f.) from three mice per time point. ( i ) Ctgf , Klf5 and Fli1 mRNA levels in the lung were assessed by qRT-PCR. n =9 mice per group. ( j ) Protein levels of CTGF, KLF5 and Fli1 in lung homogenates were assessed by immunoblotting. The results are from representative experiments that have been repeated three times in different pairs of mice with similar results. ( k ) Representative lung sections from three WT and three Klf5 +/− ; Fli1 +/− mice are shown. Pro-surfactant protein C (pro-SP-C), a specific marker for type 2 alveolar cells, is stained with FITC (green). CTGF is stained with Alexa Flour 555 (red). Nuclei are stained with 4′,6-diamidino-2-phenylindole (DAPI, blue). Scale bar, 50 μm. Data are mean±s.e.m. * P <0.05, ** P <0.01, *** P <0.001 by two-tailed Mann–Whitney U -test. The significant differences in e , h are compared with WT groups. Full size image Klf5 +/− ; Fli1 +/− mice have collagen fibril abnormalities In 2-month-old Klf5 +/− ; Fli1 +/− mice, electron microscopy delineated irregular, thickened collagen fibrils in longitudinal sections and higher fibril diameter variability in transverse sections (WT: mean, 60.8 nm; range, 34.1–92.4 nm; Klf5 +/− ; Fli1 +/− : 100.3 nm; 11.0–249.3 nm; Fig. 5i ), which are reminiscent of the findings in SSc skin [21] . In contrast, Klf5 heterozygosity only moderately increased fibril diameter and Fli1 heterozygosity just caused emergence of small diameter fibrils ( Klf5 +/− : 75.4 nm; 19.4–157.5 nm; Fli1 +/− : 62.0 nm; 11.0–105.9 nm). These observations suggest that the double heterozygous deficiency might dysregulate enzymes involved in fibrillogenesis, collagen fibril processing and assembly [22] . Interestingly, the skin of Klf5 +/− ; Fli1 +/− mice and SSc patients shared similar fibrillogenesis-associated gene expression patterns, including decreased Dcn expression and increased levels of Lum and Adamts2 ( Supplementary Fig. 8a,b ). Moreover, in cultured fibroblasts, FLI1 gene silencing decreased DCN expression, while KLF5 gene silencing increased LUM and ADAMTS2 levels ( Supplementary Fig. 8c ). These data indicate that Fli1 and KLF5 differently but coordinately regulate fibril diameter via modifying the expression of fibrillogenesis-associated molecules and that their downregulation induces an SSc-like skin phenotype at an ultrastructural level. Klf5 +/− ; Fli1 +/− mice exhibit skin vascular abnormalities Vascular injury in SSc leads to vascular structural changes [23] , reduced capillary density [24] , decreased blood flow velocity [25] and tissue hypoxia [26] . Whereas Klf5 +/− ; Fli1 +/− mice did not show macroscopic telangiectasia, ex vivo visualization of cutaneous vasculature showed vascular stenosis and bushy capillary tips in as early as 1-month-old Klf5 +/− ; Fli1 +/− mice ( Fig. 6a ). In contrast, WT and Klf5 +/− mice showed well-organized vascular structures and Fli1 +/− mice exhibited only slightly tortured vascular networks. Furthermore, histological analyses detected a progressive decrease in subcutaneous vascular density starting from 2 months of age ( Fig. 6b ). To examine dermal vascular structures in live mice, we employed multicolour two-photon in vivo imaging technique, demonstrating dense collagen accumulation and decreased vascularity in 4-month-old Klf5 +/− ; Fli1 +/− mice ( Fig. 6c ). Moreover, visualization of vascular real-time kinetics revealed reduced arteriolar blood flow velocity and interstitial hypoxia ( Fig. 6d,e ). Fli1 deficiency in endothelial cells causes vascular disintegrity [27] and CTGF induces vascular remodelling [28] , suggesting that they synergize to induce vascular abnormalities in Klf5 +/− ; Fli1 +/− mice resembling SSc vasculopathy. Lung fibrotic and vascular changes in Klf5 +/− ; Fli1 +/− mice We next examined the lung histology in Klf5 +/− ; Fli1 +/− mice because this organ frequently shows fibrotic changes in SSc. Mild thickening of alveolar septa in subpleural regions was found in 2-month-old Klf5 +/− ; Fli1 +/− mice ( Fig. 7a ). Furthermore, the loss of fine alveolar structure and increased collagen deposition were identified in 4-month-old mice ( Fig. 7c ). Strikingly, 8-month-old mice developed a diseased lung resembling human non-specific interstitial pneumonia, the main histological pattern of SSc-interstitial lung disease (ILD; Fig. 7a,b ) [29] . Diffuse uniform expansion of alveolar septa with patchy septal lymphocytic infiltration was present, while the pathological findings indicating usual interstitial pneumonia, honeycombing or fibroblastic foci were rarely seen. Moreover, we found enhanced proliferation of endothelial and vascular smooth muscle cells at 3 months of age ( Fig. 7d ) and progressive obliteration of arterioles starting from 4 months of age ( Fig. 7e ). The pulmonary arterioles finally developed markedly thickened vascular walls with expansion of α-SMA-positive cells at 8 months of age ( Fig. 7f ), simulating pathological features of pulmonary arterial hypertension [30] . Similarly, interseptal venules showed intimal fibrosis, focal luminal narrowing and perivascular lymphocytic infiltrates, all suggestive of pulmonary veno-occlusive disease ( Fig. 7g ). Pulmonary vascular beds in Klf5 +/− ; Fli1 +/− mice decreased along with the time course from 4 months of age ( Fig. 7h ). Importantly, consistent with enhanced CTGF expression in whole lung tissue ( Fig. 7i,j ), hyperplastic alveolar type 2 cells (AT2s) were positive for CTGF in Klf5 +/− ; Fli1 +/− lungs ( Fig. 7k ). Given that AT2-specific CTGF overexpression induces alveolar and vascular changes similar to Klf5 +/− ; Fli1 +/− mice [31] , CTGF induction in AT2s should contribute to SSc-ILD-like changes in Klf5 +/− ; Fli1 +/− mice. B-cell activation and autoimmunity in Klf5 +/− ; Fli1 +/− mice A large body of evidence has suggested the involvement of altered B-cell behaviour in the development of SSc [1] , [23] , [32] . While B-cell infiltration is not usually prominent in the lesional skin of SSc patients, an activated B-cell signature in SSc skin has been clearly demonstrated by DNA microarray analysis [4] . Furthermore, SSc-ILD frequently exhibits diffuse or aggregated B-cell infiltrates [33] . On the basis of these observations, we explored whether B-cell accumulation is present in the skin and lung tissue of Klf5 +/− ; Fli1 +/− mice. While the skin did not show apparently increased B-cell infiltration, Klf5 +/− ; Fli1 +/− lungs demonstrated perivascular B-cell accumulation starting from 3 months of age, which progressed to prominent B-cell lymphoid aggregates and diffuse interstitial infiltrates at 8 months of age ( Fig. 8a ) as occasionally seen in SSc-ILD [33] . The findings propose that infiltrating B cells might damage vascular and interstitial tissues in Klf5 +/− ; Fli1 +/− lungs and help induce vascular and fibrotic changes. 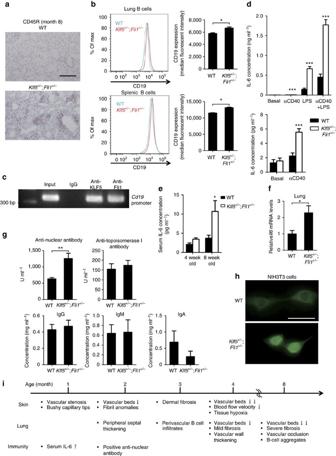Figure 8:Klf5+/−;Fli1+/−mice exhibit pulmonary infiltration of activated B cells and autoimmunity. (a) Pulmonary B cells with CD45R staining in 8-month-old mice. Scale bar, 200 μm. (b) CD19 expression in lung and splenic B cells assessed by flow cytometry. The median fluorescent intensity of CD19 expression is quantified.n=4 mice per group. (c) ChIP assay on splenic B cells assessing the binding of KLF5 and Fli1 to theCd19promoter. (d) IL-6 concentration in culture supernatants from splenic B cells stimulated for 48 h with lipopolysaccharide (LPS) and/or anti-CD40 antibody (αCD40). A total of eight duplicate cultures of cells pooled from four mice per group were examined. The data with lower concentrations are shown separately. The significant difference is compared in each pair. (e) Serum IL-6 concentration in WT andKlf5+/−;Fli1+/−mice at the ages of 4 and 8 weeks assessed by enzyme-linked immunosorbent assay (ELISA).n=7 mice per group. Significant differences are compared with the WT group in each set. (f)Il-6mRNA levels in the lung of WT andKlf5+/−;Fli1+/−mice assessed by qRT-PCR.n=7 mice per group. (g) Serum concentrations of anti-nuclear antibodies, anti-topoisomerase I antibodies (n=6 mice per group), total IgG, IgM, and IgA (n=4 mice per group) assessed by ELISA. (h) Immunofluorescent ANA assay using NIH3T3 cells. Scale bar, 50 μm. (i) The summary of SSc-like manifestations inKlf5+/−;Fli1+/−mice. Data are mean±s.e.m. *P<0.05, **P<0.01, ***P<0.001 by two-tailed Mann–WhitneyU-test. Figure 8: Klf5 +/− ; Fli1 +/− mice exhibit pulmonary infiltration of activated B cells and autoimmunity. ( a ) Pulmonary B cells with CD45R staining in 8-month-old mice. Scale bar, 200 μm. ( b ) CD19 expression in lung and splenic B cells assessed by flow cytometry. The median fluorescent intensity of CD19 expression is quantified. n =4 mice per group. ( c ) ChIP assay on splenic B cells assessing the binding of KLF5 and Fli1 to the Cd19 promoter. ( d ) IL-6 concentration in culture supernatants from splenic B cells stimulated for 48 h with lipopolysaccharide (LPS) and/or anti-CD40 antibody (αCD40). A total of eight duplicate cultures of cells pooled from four mice per group were examined. The data with lower concentrations are shown separately. The significant difference is compared in each pair. ( e ) Serum IL-6 concentration in WT and Klf5 +/− ; Fli1 +/− mice at the ages of 4 and 8 weeks assessed by enzyme-linked immunosorbent assay (ELISA). n =7 mice per group. Significant differences are compared with the WT group in each set. ( f ) Il-6 mRNA levels in the lung of WT and Klf5 +/− ; Fli1 +/− mice assessed by qRT-PCR. n =7 mice per group. ( g ) Serum concentrations of anti-nuclear antibodies, anti-topoisomerase I antibodies ( n =6 mice per group), total IgG, IgM, and IgA ( n =4 mice per group) assessed by ELISA. ( h ) Immunofluorescent ANA assay using NIH3T3 cells. Scale bar, 50 μm. ( i ) The summary of SSc-like manifestations in Klf5 +/− ; Fli1 +/− mice. Data are mean±s.e.m. * P <0.05, ** P <0.01, *** P <0.001 by two-tailed Mann–Whitney U -test. Full size image We next investigated the function of Klf5 +/− ; Fli1 +/− B cells. Importantly, CD19 functions as the dominant signalling component of a multimolecular complex on the surface of mature B cells and plays a crucial role in maintaining the balance between humoral immune response and immune tolerance [34] . Furthermore, CD19 expression has dramatic effects on B-cell activity [35] , [36] and is increased in peripheral blood B cells from SSc patients by ~20% compared with those from healthy individuals [37] . Therefore, we speculated that CD19 expression might be altered in Klf5 +/− ; Fli1 +/− B cells. In support of our hypothesis, CD19 expression was enhanced in Klf5 +/− ; Fli1 +/− B cells by 15% in the lung and by 14% in the spleen ( Fig. 8b ). Moreover, ChIP revealed that both KLF5 and Fli1 interact with the Cd19 promoter ( Fig. 8c ), suggesting that these two transcription factors intrinsically regulate Cd19 expression. A previous report indicated that CD19 expression levels are closely linked to interleukin-6 (IL-6) production from B cells [38] . B cells are an important source of IL-6 (ref. 39 ), which is capable of inducing type I collagen and CTGF [40] and is overexpressed in the skin, serum and peripheral blood mononuclear cells from SSc patients [40] , [41] . Strikingly, Klf5 +/− ; Fli1 +/− B cells produced three times greater amount of IL-6 than WT B cells in response to lipopolysaccharide and/or anti-CD40 antibody ( Fig. 8d ), consistent with elevated IL-6 levels in the serum and lung ( Fig. 8e,f ). In addition to the link with IL-6 overproduction, even a 15–29% increase in CD19 expression is known to induce autoantibody production in mice [37] , suggesting a possible induction of autoimmunity in Klf5 +/− ; Fli1 +/− mice. As expected, Klf5 +/− ; Fli1 +/− mice showed circulating anti-nuclear antibody (ANA) although total IgG, IgM, IgA or anti-topoisomerase I antibody titres were not elevated ( Fig. 8g ). Immunofluorescence assays applying sera from Klf5 +/− ; Fli1 +/− mice demonstrated nuclear staining with NIH3T3 cells in contrast to negative staining in WT mice ( Fig. 8h ). These results suggest that the partial deletion of KLF5 and Fli1 activates B cells to produce autoantibody and excessive IL-6. While several mouse models have been reported to develop cutaneous and pulmonary changes resembling SSc [42] , [43] , none have reproduced all three pathogenetic components of SSc, including vasculopathy, immune dysregulation and fibrosis [1] . Our model demonstrates a novel concept that heterozygous deficiency of two transcription factors induces the pathogenic triad. Remarkably, the natural course of the disease observed in SSc patients is also preserved in the mutant mice, with autoimmunity and vasculopathy preceding the development of skin fibrosis, then followed by progressive lung fibrosis ( Fig. 8i ). Our studies underscore the significance of epigenetic reprogramming in the pathogenesis of SSc and implicate the KLF5 and Fli1 pathways as central mediators of this disease. We demonstrated that KLF5 is epigenetically inhibited in SSc fibroblasts as is the case with Fli1 (ref. 8 ). In a certain subtype of SSc, diffuse cutaneous SSc (dcSSc), while skin sclerosis rapidly progresses at an early stage, it regresses spontaneously thereafter [44] , suggesting the involvement of a reversible phenotypic change. Furthermore, explanted SSc dermal fibroblasts continue to overproduce ECM, but this phenotype wears off with successive passages [45] . These observations suggest that reversible changes in gene expression, such as epigenetic alterations, are possibly present in dermal fibroblasts. In line with this expectation, genome-wide DNA methylation analysis in dermal fibroblast recently demonstrated a substantial number of differentially methylated genes in both dcSSc and limited cutaneous SSc [15] . Although our study and a previous report [8] clearly show the methylation of the KLF5 and Fli1 promoter regions, they were not detected in this genome-wide analysis possibly because of differences in methodology or patient population. Consistent with the evidence of aberrant methylation, cutaneous ECM overproduction in SSc is affected by epigenetic modifications, and the therapeutic potential of epigenetic modifiers has been described [14] . However, epigenetic inhibitors, such as DNA methyltransferase inhibitors and histone deacetylase inhibitors, affect a broad range of gene expressions and could have significant adverse reaction. Recently, high-throughput screening has allowed the quick discovery of drug candidates by screening a library of preexisting bioactives [46] . If a compound that specifically upregulates KLF5 and/or Fli1 expression is identified, this could have a therapeutic potential against SSc which still has no cure. SSc is categorized into three major subtypes depending on patients’ autoantibodies, for example, anti-topoisomerase I, anti-centromere and anti-RNA polymerase III antibodies. Dermal fibroblasts in patients with anti-RNA polymerase III antibody demonstrated less significant reduction in KLF5 and Fli1 expressions compared with those with anti-topoisomerase I or anti-centromere antibodies. Intriguingly, the temporal clustering of SSc and cancer has been observed in patients with autoantibodies to RNA polymerase III, but not in patients with autoantibodies to topoisomerase I or centromere, suggesting that this SSc subset may represent a distinct disease mechanism [47] , [48] . In addition to the previously identified Fli1 downregulation [49] , morphea fibroblasts also showed a significant decrease in KLF5, indicating that downregulation of these two transcription factors might be also partly responsible for localized skin sclerosis. The skin of Klf5 +/− ; Fli1 +/− mice showed a thickened dermis, increased collagen accumulation and tightly packed collagen fibres, resembling the dermal changes frequently seen in SSc patients [1] . Although KLF5 itself was found to be a potent transcriptional repressor of CTGF, its heterozygous deficiency or fibroblast-specific depletion alone did not induce skin fibrosis unless other triggers, such as bleomycin or the tsk phenotype, were included. This appears reasonable because CTGF overexpression [50] or KLF5 deficiency [10] , [11] usually requires additional triggering stimuli to develop tissue fibrosis in other organs. Importantly, Fli1 plays a pivotal role in the regulation of ECM genes [22] , [51] , [52] , and thus its downregulation and the subsequent upregulation of ECM genes should coordinately work with further CTGF overproduction induced by simultaneous downregulation of KLF5 and Fli1, plausibly leading to spontaneous dermal fibrosis in Klf5 +/− ; Fli1 +/− mice. In addition to CTGF and collagens, pro-fibrotic genes that are characteristically upregulated in SSc skin, such as Fn1 and Tsp1 (refs 4 , 53 ), showed significantly higher expression in the skin of Klf5 +/− ; Fli1 +/− mice while Comp expression, which is enhanced and moderately correlates with the severity of skin sclerosis in SSc [54] , was not significantly increased in Klf5 +/− ; Fli1 +/− skin. The discrepancy in Comp gene expression could be caused by the differences in species, or might be explained by a phenotypical difference between dcSSc patients and Klf5 +/− ; Fli1 +/− mice. Considering that the skin gene expression pattern largely recapitulates features of SSc, investigating the skin phenotype of Klf5 +/− ; Fli1 +/− mice could clarify the pathogenic mechanism of SSc and reveal new treatment targets. Klf5 +/− ; Fli1 +/− mice and SSc patients also shared common alterations in collagen fibril structure and expression of fibrillogenesis-associated molecules. Fibril assembly is mediated by collagen-processing enzymes and also modified by small leucine-rich repeat proteoglycans [55] . The knockout of small leucine-rich repeat proteoglycans, such as decorin, biglycan, lumican and fibromodulin, causes fibril diameter abnormalities [56] , [57] , [58] . Our in vitro data suggest that reduced decorin expression is primarily attributed to Fli1 downregulation, while increased lumican and ADAMTS2 (a disintegrin and metalloproteinase with thrombospondin motifs 2) expressions are attributable to KLF5 downregulation. Importantly, although Fli1 heterozygous deficiency caused only a slight change in fibril diameter, it significantly amplified the fibril change induced by Klf5 heterozygous deficiency, suggesting that Fli1 and KLF5 have distinct roles in fibril diameter regulation and coordinately regulate fibrillogenesis-associated genes. Furthermore, similar to SSc patients [23] , [24] , [25] , [26] , Klf5 +/− ; Fli1 +/− mice developed vascular structural changes, reduced vascular density, decreased blood flow and interstitial hypoxia in the skin. Vascular networks of Klf5 +/− mice are apparently normal and those of Fli1 +/− mice demonstrated only a modest morphological change, clearly showing that simultaneous disruption of these two transcriptional factors induces far more significant vascular abnormalities compared with single heterozygous deficiency. Given that endothelial cell-specific deletion of Fli1 elicits substantial structural changes in peripheral vasculature [27] , Fli1 heterozygosity should be partially responsible for the strikingly disorganized vasculature in Klf5 +/− ; Fli1 +/− mice. Notably, periadventitial administration of recombinant CTGF induces neointimal thickening, enlargement of an external elastic lamina area, adventitial collagen accumulation, adventitial myofibroblast transformation and proliferation of vascular wall cells [28] . Therefore, CTGF overproduction in the skin tissue of Klf5 +/− ; Fli1 +/− mice could possibly work together with Fli1 reduction, leading to an altered vascular system. The peak onset of SSc is between the ages of 40 and 50 (ref. 59 ) and lung lesions often fully develop years later, which corresponds with the late onset of full-blown SSc-like lung abnormalities in Klf5 +/− ; Fli1 +/− mice. Interstitial fibrosis and alveolar architectural changes progressed with the time course, and Klf5 +/− ; Fli1 +/− lungs eventually developed arterial and venous occlusion. The non-specific interstitial pneumonia-like interstitial changes and pulmonary veno-occlusive disease-like venous involvement in Klf5 +/− ; Fli1 +/− mice strongly suggest a common aetiology shared between SSc-ILD and Klf5 +/− ; Fli1 +/− lungs because both of these findings are characteristic of SSc lungs [29] , [60] . In pulmonary fibrosis, CTGF has a critical role as shown by the effectiveness of anti-CTGF therapy in experimental lung fibrosis models [6] and increased CTGF gene expression in SSc lung tissues [61] . Furthermore, the conditional overexpression of CTGF in AT2s induces alveolar and vascular changes similar to Klf5 +/− ; Fli1 +/− mice [31] . Thus, CTGF induction in AT2s by downregulation of KLF5 and Fli1 emerges as a key event that triggers pulmonary interstitial fibrosis and vascular alterations. In Klf5 +/− ; Fli1 +/− mice, the lung showed prominent B-cell infiltrates, and B cells demonstrated functional changes characterized by increased CD19 expression and IL-6 overproduction. The clinical significance of B cells and IL-6 in SSc is described by recent preliminary studies showing that SSc manifestations are relieved in a certain subset of patients by tocilizumab [62] , an anti-IL-6 receptor antibody and rituximab [63] , an anti-B-cell therapy. Similar to the Klf5 +/− ; Fli1 +/− lung, SSc-ILD frequently shows diffuse or aggregated B-cell infiltrates [33] . CD19 expression is increased in peripheral blood B cells from SSc patients by ~20% compared with healthy individuals [37] . Moreover, IL-6 serum levels correlate with skin fibrosis severity and prognosis of SSc patients [40] , [64] . As for autoimmunity, while we did not detect autoantibodies reacting to topoisomerase I, Klf5 +/− ; Fli1 +/− mice demonstrated positive for ANA. Taken together, heterozygous deficiency of KLF5 and Fli1 activates B cells and induces autoimmunity, possibly interplaying with vascular and fibrotic alterations, and leading to the establishment of SSc-like manifestations in Klf5 +/− ; Fli1 +/− mice. In summary, Klf5 +/− ; Fli1 +/− mice share principal manifestations of SSc, including tissue fibrosis, vasculopathy and immune activation. Thus, Klf5 +/− ; Fli1 +/− mice represent a novel genetic animal model of SSc based on partial deletion of two transcription factors, which are expressed at reduced levels in SSc skin. In SSc, epigenetic mechanisms contribute to suppression of KLF5 and Fli1, at least in dermal fibroblasts. Our study suggests a novel concept that the downregulation of these two transcription factors is the primary event triggering the three major manifestations in SSc. This new model should be helpful in better understanding the pathogenesis of SSc, which currently has no therapy capable of reversing the progression. Patients and fibroblast cultures Human skin samples were taken from the forearm of 8 dcSSc patients (seven with anti-topoisomerase I antibody and one without ANA) having skin sclerosis for less than 2 years. All of the patients were diagnosed with clinical appearance and histological findings, and none of them had any other collagen diseases. Control fibroblasts were obtained by skin biopsy from sex- and site-matched eight healthy donors with closely matched age. Institutional approval (University of Tokyo Graduate School of Medicine) and written informed consent were obtained from all the subjects. Fibroblasts were cultured in minimum essential medium with 10% fetal bovine serum (FBS), 2 mM L -glutamine and antibiotic–antimycotic solution. These cells were individually maintained as monolayers at 37 °C in 95% air and 5% CO 2 . All studies used cells from passage number 3 to 6. Animal models We generated Klf5 +/− and Klf5 fl/fl mice with the C57Bl/6J (B6) background using plasmid-targeting vectors [10] , [12] . Fli1 +/− mice were kindly provided by Dennis K. Watson [13] . Tsk/+ (014632, B6.Cg- Fbn1 Tsk /J) and Col1a2-Cre (016237, B6.Cg-Tg(Col1a2-cre/ERT)7Cpd/J) mice were purchased from Jackson Laboratory. To induce fibroblast-specific KLF5 deletion, Klf5 fl/fl ; Col1a2-Cre/ERT mice had intraperitoneal injections of 1 mg of tamoxifen dissolved in corn oil for five consecutive days starting from 3 weeks of age. Klf5 −/− or Fli1 −/− mice die in utero [12] , [13] . All experiments were approved by the University of Tokyo Ethics Committee for Animal Experiments and strictly adhered to the guidelines for animal experiments of the University of Tokyo. Skin fibrosis was induced in 6-week-old female Klf5 +/− or Klf5 fl/fl ; Col1a2-Cre/ERT mice by subcutaneous injections of bleomycin to the back skin every other day for 3 weeks. Male mice were used when we assessed skin abnormalities in Klf5 +/− ; Fli1 +/− mice. The age of mice is often specified in each study, but 8- to 16-week-old sex-matched mice were utilized unless otherwise mentioned. We performed animal studies at least twice. Collagen measurement Following the instruction of QuickZyme Total Collagen Assay (QZBtotcol, QuickZyme, Leiden, Netherlands), skin and lung tissues were hydrolyzed with 6 N HCl for 20 h at 95 °C, and total collagen content was quantified. Six-mm punch biopsy skin samples and total left lobes of the lung were used. Enzyme-linked immunosorbent assay Mouse sera were analysed by the following enzyme-linked immunosorbent assay kits: mouse ANA, mouse anti-topoisomerase I antibody (5210 and 6110; Alpha Diagnostic International, San Antonio, TX, USA), mouse total IgG, IgM, and IgA (88-50400, 88-50470, and 88-50450; eBioscience, San Diego, CA, USA), and mouse IL-6 (M6000B, R & D Systems, Minneapolis, MN, USA). Reagents Anti-KLF5 (KM1784, KM3918) antibody was described previously [10] , [11] . KM1784 was used for immunohistochemistry (1/200), while KM 3918 was used for in vitro assays (1/1,000 dilution). Anti-CTGF (1/100 dilution, sc-14939), anti-Fli1 (1/1,000 dilution, sc-356) and anti-Ets1 (1/1,000 dilution, sc-111) antibodies were purchased from Santa Cruz Biotechnology (Santa Cruz, CA, USA). Anti-α-SMA (1/1,000 dilution, A2547) and anti-β-actin (1/2,000 dilution, A5441) antibodies were from Sigma-Aldrich (St Louis, MO, USA). Anti-Fli1 antibody for immunohistochemistry was from R&D (1/50 dilution, AF6474). Anti-acetyl histone H3 and H4 (1/1,000 dilution, 06-599 and 06-866), anti-pro-surfactant protein C (AB3786) and anti-von Willebrand factor (1/100 dilution, AB7356) antibodies were from EMD Millipore Corporation (Billerica, MA, USA). Anti-type I collagen antibody (1/1,000 dilution, 1310-01) was from Southern Biotech (Birmingham, AL, USA). Anti-proliferating cell nuclear antigen antibody (1/4,000 dilution, ab18197) was purchased from Abcam (Cambridge, UK). Anti-Smad3 (1/1,000 dilution, 9523), anti-phospho-smad3 (1/1,000 dilution, 9520), anti-ERK (1/1,000 dilution, 4695), anti-phospho-ERK (1/1,000 dilution, 4370), anti-p38 (1/1,000 dilution, 9212), anti-phospho-p38 (1/1,000 dilution, 9211), anti-JNK (1/1,000 dilution, 9258) and anti-phospho-JNK (1/1,000 dilution, 4671) antibodies were purchased from Cell Signaling Technology (Danvers, MA, USA). Immunohistochemistry Human and mouse samples were fixed in formalin, dehydrated, embedded in paraffin and sectioned. Vectastain ABC kit (Vector Laboratories, Burlingame, CA, USA) was used according to manufacturer’s instruction. Regarding human studies in Fig. 4 , skin samples from five healthy individuals and five patients with each following disease or disease subtype were used: dcSSc with an anti-topoisomerase I antibody, limited cutaneous SSc with an anti-centromere antibody, dcSSc with an anti-RNA polymerase III antibody, morphea and eosinophilic fasciitis. As for mouse studies, the back skin and the right lower lobe of the lung were harvested. Skin thickness and cell counts were scored by S. Noda. and Y.A. in at least randomly chosen five high power fields of samples and the average number for each sample was used. Each section was examined independently in a blinded fashion. FITC-conjugated anti-rabbit (sc-2090, Santa Cruz) and Alexa Fluor 555-conjugated anti-goat (A21432; Life Technologies, Carlsbad, CA, USA) were used for immunofluorescence studies as secondary antibodies at a 1/200 dilution. ANA detection ANA was detected by indirect immunofluorescence methods using NIH3T3 cells (CRL-1658, American Type Culture Collection, Manassas, VA, USA). Murine sera (1/160 dilution) were incubated on the slides, followed by detection with FITC-labeled anti-mouse IgG (AP308F, Millipore, 1/100 dilution). Transmission electron microscopy Samples were obtained from the back skin of 2-month-old mice of each strain, fixed, postfixed, rinsed, dehydrated, transferred to propylene oxide and embedded in epoxy resin. Ultra-thin sections were stained with tannate, uranyl acetate and lead citrate and examined with a JEM-1200EX (JEOL, Tokyo, Japan). Multiple micrographs of cross-sections of dermal collagen fibrils were chosen randomly and used for morphometry. Mean diameter, range and frequency distribution profiles were obtained by manually measuring the smallest diameter of 500 collagen fibrils. Immunoblotting Confluent quiescent fibroblasts were serum starved for 24 h. Whole cell lysates and nuclear extracts were prepared. Skin and lung samples from mice were homogenized in RIPA Lysis Buffer (sc-24948, Santa Cruz) and the supernatants after centrifugation were used. Samples were subjected to SDS–polyacrylamide gel electrophoresis (Life Technologies) and immunoblotting with antibody dilution of 1/1,000. Bands were detected using enhanced chemiluminescent techniques (Thermo Fisher Scientific, Rockford, IL, USA). The following secondary antibodies were used at a 1/1,000 dilution: anti-mouse IgG-HRP, anti-rabbit IgG-HRP (sc-2371 and sc-2955, Santa Cruz) and anti-goat IgG-HRP (55363; MP Biomedicals, Santa Ana, CA, USA). MagicMark XP Western Protein Standard (LC5602, Life Technologies) or Precision Plus Protein Dual Color Standards (161-0374; Bio-Rad, Hercules, CA, USA) was used for molecular weight confirmation. Full blotting images are shown in Supplementary Fig. 9 . Small interfering RNA Cells were transfected with KLF5 siRNA (ON-TARGETplus SMARTpool, L-013571-00-0005, Thermo Fisher Scientific), Fli1 siRNA (sc-35384, Santa Cruz) or control scrambled RNA (sc-37007, Santa Cruz) for 24 h using HiPerFect Transfection Reagent (301705, Qiagen, Hilden, Germany) shortly after seeding. Thereafter, cells were serum starved for 24 h and subsequently harvested. RNA isolation and qRT-PCR RNA (1 μg) was extracted using RNeasy Mini Kit (74104, Qiagen) or RNeasy Fibrous Tissue Mini Kit (74704, Qiagen) and reverse-transcribed using iScript cDNA Synthesis Kits (170-8891, Bio-Rad). qRT-PCR was carried out using Fast SYBR Green PCR Master Mix (4385617, Life Technologies) or TaqMan Universal PCR Master Mix (4304437, Life Technologies) on ABI prism 7000 (Life Technologies) in triplicates. The mRNA levels were normalized to those of 18S rRNA gene. The sequences of the primers used are shown in Supplementary Table 1 except for Comp (Mm00489490_m1, Life Technologies). Dissociation analysis for each primer pair and reaction was performed to verify specific amplification. ChIP assay The ChIP assay was carried out using EpiQuik ChIP kit (P-2002; Epigentek, Farmingdale, NY, USA). In brief, cells were treated with 1% formaldehyde. The crosslinked chromatin was then prepared and sonicated to an average size of 300–500 bp. The DNA fragments were immunoprecipitated with the indicated antibodies. As a negative control, normal rabbit or mouse IgG was used. Input corresponds to extracted DNA from the sample before immunoprecipitation. After reversal of crosslinking, the immunoprecipitated chromatin was analysed by agarose gel electrophoresis and qRT-PCR. The results of qRT-PCR were normalized to input values. The primers amplifying the proximal promoter regions of human KLF5 or CTGF genes were used. The sequences of the PCR primers were as follows: the human KLF5 promoter, 5′- CAGCCCAATCTGTCAGAGAAGT -3′ and 5′- CGCCTCTATTTCACCCAACTC -3′; the human CTGF promoter containing the KBE1 sequence, 5′- TCCGGTGTGAGTTGATGAGG -3′ and 5′- GCGGGGAAGAGTTGTTGTGT -3′; the mouse Cd19 promoter, 5′- GGAAAGCTCTGTGTGTGCAGT -3′ and 5′- GGAGAGGAGATGGCATGGTAG -3′. Full images of gel electrophoresis are shown in Supplementary Fig. 9 . Bisulfited DNA sequencing Genomic DNA was isolated from cultured normal and SSc fibroblasts using NucleoSpin Tissue (740952; Macherey-Nagel, Düren, Germany). Bisulfite modification was performed using MethylEasy Xceed Rapid DNA Bisulphite Modification Kit (ME002; Human Genetic Signatures, North Ryde, Australia). Purified bisulfite-modified DNA was amplified using EpiTaq HS (R110A, Takara Bio, Kyoto, Japan). Primers were designed using MethPrimer ( http://www.urogene.org/methprimer ) to amplify a sequence including 4 CpG islands of the KLF5 promoter on the nucleotides from −273 to −210. The primer sequences are 5′- TTGTTAGAGAAGTTGTGTATAAATTG -3′ and 5′- ACCAACCTATAAACAAAAAAAA -3′. The amplified PCR products were ligated into pMD20T-vector using Mighty TA-cloning Kit (6028, Takara Bio) and amplified in transformed bacteria Escherichia coli (9128, HST08, Takara Bio). Sequencing was completed by Takara Bio. The primer for sequencing of bisulfited KLF5 promoter was the M13 primer RV, 5′- CAGGAAACAGCTATGAC -3′. QUMA ( http://quma.cdb.riken.jp ) was used for methylation analyses. Plasmids A fragment of the CTGF promoter (−823 to +74) cloned into the cloning site of pGL2-basic vector was a gift from Dr Gary Grotendorst [65] . pCAG-KLF5 was generated by inserting KLF5 cDNAs into pCAGMS [66] . pSG5-Fli1 was kindly provided by Dennis K. Watson [67] . QuikChange II Site-Directed Mutagenesis Kit (200523, Agilent Technologies, Santa Clara, CA, USA) was used to generate site-directed mutant CTGF promoter constructs. Plasmid vectors were amplified in transformed bacteria Escherichia coli (9057, DH5α, Takara Bio) and isolated using Plasmid Midi Kit (12145, Qiagen). Reporter gene assay Human foreskin fibroblasts were transfected with plasmids using X-tremeGENE 9 DNA Transfection Reagent (06365787001; Roche, Basel, Switzerland). Lipofectamine 2000 (11668019, Life Technologies) was used for the cotransfection of plasmids and siRNA. The cells were harvested after 30 h, and the activities of both firefly luciferase and Renilla luciferase were measured with AB-2200 luminometer (ATTO, Tokyo, Japan) using dual luciferase reporter system (E1910; Promega, Madison, WI, USA). The activity of firefly luciferase was normalized to that of Renilla luciferase (E2241, Promega). A minimum of three independent transfections was performed for each experimental group. Oligonucleotide pull-down assay The oligonucleotides containing biotin on the 5′ nucleotide of the sense strand were used. The sequences of these oligonucleotides were as follows: (i) CTGF KBE1 oligonucleotides, 5′- GAGGCAGGAA GGTGGGGAG GAATGCGAGGAATGTCCCTGTTTGTG -3′ and 5′- CACAAACAGGGACATTCCTCGCATTCCTCCCCACCTTCCTGCCTC -3′, which correspond to base pairs −123 to −79 of the CTGF promoter containing KBE1; (ii) CTGF mutated KBE1 oligonucleotides, 5′- GAGGCAGGAA GGTAAAGAG GAATGCGAGGAATGTCCCTGTTTGTG -3′ and 5′- CACAAACAGGGACATTCCTCGCATTCCTCTTTACCTTCCTGCCTC -3′, which have mutated KBE1; (iii) CTGF KBE2 oligonucleotides, 5′- TAGGA CTCCA TTCAGCTCATTGGCGAGCCGCGGCCGCCCG -3′ and 5′- CGGGCGGCCGCGGCTCGCCAATGAGCTGAATGGAGTCCTA -3′, which correspond to base pairs −78 to −39 of the CTGF promoter containing KBE2; and (iv) CTGF KBE3 oligonucleotides, 5′- GAGTGTGCCAGCTTTTTCAGAC GGAG GAATGCTGAGTGTCAAG -3′ and 5′- CTTGACACTCAGCATTCCTCCGTCTGAAAAAGCTGGCACACTC -3′, which correspond to base pairs −195 to −153 of the CTGF promoter containing KBE3. These oligonucleotides were annealed to their respective complementary oligonucleotides at 95 °C for 1 h (ref. 68 ). Nuclear extracts prepared from dermal fibroblasts from healthy individuals were incubated with streptavidin-coupled agarose beads and 500 pmol of each double-stranded oligonucleotide for 2 h at room temperature with gentle rocking. The protein–DNA–streptavidin–agarose complex was washed four times with PBS containing protease inhibitors. The precipitates were subjected to immunoblotting using the indicated antibodies. Immunoprecipitation To precipitate endogenous Fli1 or Ets1 in dermal fibroblasts from healthy individuals, we used Pierce Crosslink IP Kit (26147, Thermo Fisher Scientific) as per manufacturer’s instructions. In brief, the indicated antibodies for immunoprecipitation were incubated with protein A/G for 1 h at room temperature, and then crosslinking reaction was made for 1 h at room temperature. Nuclear extracts precleared with agarose resin for 1 h at 4 °C were incubated with the antibody-crosslinked resin overnight at 4 °C. The antigens were eluted and subjected to immunoblotting. Visualization of subcutaneous vascular network Mice were anaesthetized by ethyl ether and 200 μl of FITC-conjugated dextran (2,000 kDa, 20 mg ml −1 in PBS; FD2000S, Sigma-Aldrich) was injected into the tail vein through a 28-gauge needle. After 5 min, the mice were killed and a full thickness piece of back skin (4 × 2 cm) was prepared. The skin specimen was placed directly on the slide (epidermis side up) and the structure of vascular network in the skin was visualized by fluorescence microscopy. B-cell sorting and stimulation B cells were isolated by CD19 positive selection, using MACS magnetic beads (130-052-201, Miltenyi Biotec, Bergisch Gladbach, Germany). The B-cell purity was confirmed by double staining of CD19 and CD45R using fluorescence-activated cell sorting. The 10 5 cells per well were stimulated with 5 μg ml −1 lipopolysaccharides (LPS; L5293, Sigma-Aldrich) and/or 10 μg ml −1 anti-CD40 antibody (102810, BioLegend, San Diego, CA, USA). Supernatants were harvested 48 h later. In vivo imaging To visualize vascular dynamics in the mouse skin, we used in vivo multiphoton microscopy, which was a modification of conventional single photon methods [69] . Mice were anaesthetized by injection with urethane (1.5 g kg −1 ), and they were secured to the heated stage (Tokai Hit, Fujinomiya, Japan) of an inverted microscope (Nikon, Eclipse Ti, Tokyo, Japan). Texas-Red-dextran (D1830, 25 mg kg −1 BW, 70 kDa, Life Technologies) and Hoechst 33342 (H1399, 10 mg kg −1 , Life Technologies) were injected into the mice to visualize cell dynamics and blood flow. The tissue was excited at a wavelength of 860 nm using a Ti: sapphire laser (Visio II, Coherent, Santa Clara, CA, USA), and images were captured using a Nikon A1R-MP system as XYZ-T images. Z stacks were usually ~50 μm thick with 1-μm slice images. A × 40 (N.A. 1.15) water immersion objective lens (Nikon) was used, and the images were captured at × 1.5 zoom. Some sequential images were collected for 1 min at a frame rate of 30 XY images s −1 . More than five animals were examined in each group. Images were analysed using NIS-Elements software (Nikon). Intravital microscopy and hypoxia visualization To visually analyze hypoxia within skin interstitial spaces in living animals, we modified an in vivo imaging technique using a phosphorescent hypoxia probe [70] . Hypoxia probe (LOX-1, SCIVAX, 1 mg kg −1 ), FITC-dextran (150 kDa, Sigma, FD150, 20 mg kg −1 ) and Hoechst 33342 (10 mg kg −1 , Invitrogen) were injected into anaesthetized mice. The tissue was excited at a wavelength of 920 nm using a Ti: sapphire laser (Vision II, Coherent, Santa Clara, CA) and images were captured using a Nikon A1R-MP system as XYZ-T images. Z stacks were 50 μm thick with 1-μm slice images. A × 40 (N.A. 1.15) water immersion objective lens (Nikon) was used and the images were captured at × 1.5 zoom. The phosphorescent intensity was analysed in randomly selected regions of interest using NIS-Elements software (Nikon) by blinded observers. Flow cytometry We killed the mice after general anaesthesia with systemic heparinization. We removed the lung and spleen, and then minced the lung into small pieces. We incubated them for 25 min for the lung in collagenase solution (2 mg ml −1 of collagenase type 2; LS004176; Worthington, Lakewood, NJ, USA) in 50 ml of Tyrode buffer (containing 137 mM NaCl, 5.4 mM KCl, 1.8 mM CaCl 2 , 0.5 mM MgCl 2 , 0.33 mM NaH 2 PO 4 , 5 mM HEPES and 5 mM glucose) with gentle stirring. We then filtered the samples through a 1-mm mesh. Dulbecco’s modified Eagle’s medium (30 ml) was added to each digested sample and centrifuged at 3,500 r.p.m. for 5 min. We resuspended the resultant pellet into 40 ml of Dulbecco’s modified Eagle’s medium and filtered it through a 70-μm mesh. The samples were centrifuged at 3,500 r.p.m. for 5 min again. We also processed the spleen and obtained the cell pellet. We then incubated the cell fractions for 8.5 min in erythrocyte-lysing buffer (555899, BD Biosciences, San Jose, CA, USA) in a dark room, and we finally resuspended them in PBS supplemented with 3% FBS and washed them twice. After counting the cell numbers, Fc block was performed with anti-CD16/CD32 antibody (553141, BD Biosciences, 1/1,000 dilution). We incubated these isolated cells with anti-mouse CD45R (FITC, 553088, BD Biosciences) and anti-mouse CD19 (PE/Cy7, 115519, Biolegend) at a 1/100 dilution. The cells were analysed by flow cytometry with a FACSCanto II (BD Biosciences) and FlowJo (Tree Star, Ashland, OR, USA). We used propidium iodide (P3566, Life Technologies) to exclude dead cells. Statistical analysis Statistical analysis was carried out using Prism 5 (GraphPad, La Jolla, CA, USA). Significance was calculated using a Mann–Whitney U -tests or one-way analysis of variance with Bonferroni’s post hoc test for comparison of groups greater than two. For comparing two group values that followed Gaussian distribution, two-tailed t -test was used. P <0.05 was considered statistically significant. Within-group distributions are expressed as mean±s.e.m. Sample sizes were dependent on the variation and mean of the samples. The smallest possible size of samples was employed. We did not exclude samples or animals. No formal randomization was performed. Only histopathological studies were blinded. For every figure, statistical tests are justified as appropriate. All data meet the assumptions of the tests. How to cite this article: Noda, S. et al . Simultaneous downregulation of KLF5 and Fli1 is a key feature underlying systemic sclerosis. Nat. Commun. 5:5797 doi: 10.1038/ncomms6797 (2014).